Endoplasmic reticulum stress sensitizes cells to DNA damage-induced apoptosis through p53-dependent suppression of p21CDKN1A Endoplasmic reticulum (ER) stress occurs in poorly perfused tissues and activates the p53 isoform p53/47 to promote G2 arrest via 14-3-3σ. This contrasts with the p21 CDKN1A -dependent G1 arrest caused by p53 following DNA damage. It is not known how cells respond to conditions when both pathways are activated. Here we show that p53/47 prevents p53-induced p21 transcription during ER stress and that both isoforms repress p21 mRNA translation. This prevents p21 from promoting COP1-mediated 14-3-3σ degradation and leads to G2 arrest. DNA damage does not result in p53-dependent induction of p21 during ER stress and instead results in an increase in p53-induced apoptosis. This illustrates how p53 isoforms target an intrinsic balance between the G1 and G2 checkpoints for cell cycle coordination and demonstrates an ER stress-dependent p53 pathway that suppresses p21 and lowers the apoptotic threshold to genotoxic drugs. In solid tumours, low vascularization exposes actively dividing cells to nutrient deprivation and hypoxia that affect the endoplasmic reticulum (ER) function in the folding and maturation of secretory and transmembrane proteins. An accumulation of unfolded proteins results in activation of the unfolded protein response (UPR) that either aims to restore ER homeostasis via a reduction in global protein synthesis and activation of chaperones and degradation processes, or can trigger programmed cell death under prolonged stress [1] , [2] . ER stress has been linked to numerous pathological conditions, including neurodegenerative disorder, diabetes, ischaemia and inflammation [3] . Activation of the UPR pathway can also have opposing roles in tumorigenesis and has been implicated in both aggressive tumour growth and in cancer cell death [4] , [5] , [6] . In addition, the UPR was found to alter the response of solid tumour cells to chemotherapies, with improved sensitivity or increased resistance to different genotoxic drugs [4] , [7] , [8] , [9] , [10] . However, how the DNA damage-induced stress pathway functions during the UPR remains unclear. Activation of the p53 tumour-suppressor protein in response to cellular stresses and damages serves to arrest cells in different phases of the cell cycle where the appropriate repair can take place or to induce irreversible senescence or apoptosis. These various cell biological effects are mediated by changes in the expression profile of a vast number of p53 target genes. However, it is yet relatively unknown how the activity of p53 downstream factors is synchronized to ensure that the cellular response matches the inflicting damage. The p53 gene encodes various p53 isoforms, each with its own unique activity that help to diversify p53 function in response to different signalling pathways [11] , [12] , [13] , [14] , [15] . The p53/47 isoform, later called ΔNp53 or Δ40p53, lacks the first 40 amino acids of the full-length p53 (p53 FL) and has different activity and stability [16] , [17] , [18] , [19] . UPR activation of the PERK kinase leads to eIF2α phosphorylation and a global reduction in cap-dependent translation, whereas some mRNAs required for the ER stress response are induced by PERK activity [20] , [21] , [22] . The p53 is one such mRNA and the selective PERK-dependent induction of p53/47 translation is required for 14-3-3σ-mediated G2 arrest [23] , [24] . This stop in cell cycle progression at the G2/M transition, when cap-dependent mRNA translation is naturally suppressed, favours repair to the ER [25] . p53/47 forms oligomers more easily as compared with p53 FL and relatively small changes in p53/47 levels during ER stress impose a dominant phenotype [23] . Genomic profiling has implicated p53/47 in differentiating p53 transactivation and more recent data have, in addition to cell cycle control, linked p53/47 activity to the mammalian target of rapamycin metabolic pathway and mitochondria [16] , [23] , [26] . Recent studies also identified p53/47 expression in glioblastoma and suggested a role for p53/47 in ageing and stem cell pluripotency [27] , [28] . 14-3-3 sigma (14-3-3σ) belongs to the conserved and ubiquitously expressed 14-3-3 family and regulates important cellular processes including proliferation, differentiation, cell growth and apoptosis [29] , [30] , [31] . 14-3-3σ was identified as a p53 target gene that promotes G2 arrest by sequestering the cyclin B1/CDC2 complex in the cytoplasm to prevent mitotic catastrophe upon DNA damage [32] , [33] . Loss of 14-3-3σ is observed in human cancers and has been linked to methylation of 5′CpG islands or to the E3 ligases estrogen-responsive finger protein and constitutive photomorphogenic 1 (COP1) that target 14-3-3σ for ubiquitin-dependent degradation [34] , [35] . Focal deletions of COP1 in human cancers and knockout mouse models support a role for COP1 in preventing cancer development [36] , [37] . However, elevated COP1 expression has also been reported in various human cancers and COP1 was reported to promote p53 degradation [38] , [39] . COP1 activity is regulated on the level of expression through the control of self-ubiquitination and cytoplasmic-related degradation or via controlling its substrate specificity [35] , [40] , [41] , [42] . p21 CDKN1A (p21Cip1/Waf1) is induced by p53 early in response to DNA damage and forms an important component of the p53 tumour-suppressor activity [43] . p21 knockout mice show increased tumour development at late age [44] , [45] and clinical studies have identified loss of p21 with a negative prognosis that correlates with tumour progression [46] , [47] . p21 growth-suppressor role is primarily attributed to its capacity to inhibit cyclin/cyclin-dependent kinase (CDK) complexes, thereby stopping cell cycle progression. The foremost effect of p21 is at the G1 and S phases via suppression of the cyclin E/CDK2 and cyclin A/CDK2 activity, respectively. However, induced levels of p21 have instead been linked to different types of human cancers and the incidence of radiation-induced tumours is decreased in p21-deficient animals [48] , [49] , [50] , [51] . Depending on post-translational modifications and cellular localization, p21 can support G2/M transition via activation of the cyclin B1/CDC2 or exhibit anti-apoptotic activity [52] , [53] , [54] . The regulation of p21 levels via transcription and protein stability are better known as compared with its rate of synthesis. However, several cellular factors target the 3′ untranslated region of p21 to control its mRNA stability [55] , [56] . As the UPR and DNA damage responses are simultaneously activated in cells suffering from ischaemic conditions and genomic stress, such as in genomically unstable and poorly perfused tumours and/or after genotoxic treatment, we were interested to learn how these two opposing p53 pathways are coordinated under such conditions. We show that during the UPR p53 actively suppresses p21 expression in order to allow activation of 14-3-3σ and this leads to a lowered apoptotic threshold upon DNA damage. These results reveal a p53 pathway based on the suppression of p21 and an intrinsic balance between two p53 downstream G1 and G2 regulatory factors as well as illustrate how the cellular microenvironment can affect the genomic integrity with important implications for predicting the therapeutic response to genotoxic treatments. p53-dependent suppression of p21 during ER stress Stress to the ER caused by blocking the calcium flux over the ER membrane using thapsigargin (100 nM for 16 h) triggers the UPR as shown by the induction of the ER homeostasis central regulator BiP chaperone ( Fig. 1a ). ER stress promotes cap-independent translation of p53/47 via activation of the PERK kinase and in line with this we observed an induction of p53/47 in HCT116 and A549 cells expressing endogenous p53. At the same time, we observed a reduction in the levels of p53 full-length (p53 FL) because of PERK-mediated suppression of cap-dependent translation ( Fig. 1a ). G2 arrest following ER stress requires p53/47 activity and the induction of 14-3-3 sigma (14-3-3σ) [16] , [23] , whereas G1 arrest induced by p53 FL is mediated by p21 CDKN1A (p21). In HCT116 and A549 cells, the levels of p21 expression were reduced during ER stress ( Fig. 1a ). This was not observed in the p53-negative cells H1299 and Saos-2, indicating that PERK activity does not affect p21 expression per se ( Fig. 1a ). However, when we introduced p53 wild-type cDNA that encodes both p53 isoforms in H1299 and Saos-2 cells, we observed a reduction in p21 expression with an increase in p53/47 following treatment with thapsigargin. In these transfected cells, the levels of p53 FL remained high during ER stress, indicating that the levels of p53/47, and not full-length p53, are related to the suppression of p21. Furthermore, a reduction in expression of p53 isoforms using small interfering RNA (siRNA) was sufficient to prevent ER stress-mediated suppression of p21 in HCT116 cells ( Fig. 1a ). 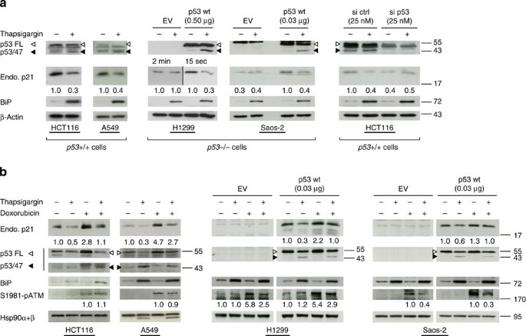Figure 1: Endoplasmic reticulum (ER) stress suppresses p21 in a dominant p53-dependent manner. (a) p53-proficient HCT116 and A549 cells or p53-deficient H1299 and Saos-2 cells transfected, or not, with p53 cDNA were treated with 100 nM thapsigargin for 16 h to induce ER stress and the unfolded protein response (UPR) or with 0.1% DMSO. Thapsigargin treatment results in an increase in p53/47 and lowered p21CDKN1A(p21) levels. Suppressing p53 isoforms by siRNA prevents the ER stress-associated decrease of p21 in HCT116 cells. (b) Treatment of cells with a 1 μM doxorubicin pulse (see Methods) induces DNA damage and activates the ATM kinase, as determined using a phosphospecific serine 1981 antibody (S1981-pATM). Inaandb, cell lysates were analysed by western blot analysis. ACMDD serum was used to detect endogenous p53 isoforms levels in HCT116 and A549 (see Methods). BiP was used as a positive control for UPR activation and β-actin or Hsp90α+β as a loading control. Numbers shown below the bands represent p21 or S1981-pATM quantification. Blots representn≥3. EV stands for empty vector and p53 FL for full-length p53 (see alsoSupplementary Fig. 1). Figure 1: Endoplasmic reticulum (ER) stress suppresses p21 in a dominant p53-dependent manner. ( a ) p53-proficient HCT116 and A549 cells or p53-deficient H1299 and Saos-2 cells transfected, or not, with p53 cDNA were treated with 100 nM thapsigargin for 16 h to induce ER stress and the unfolded protein response (UPR) or with 0.1% DMSO. Thapsigargin treatment results in an increase in p53/47 and lowered p21 CDKN1A (p21) levels. Suppressing p53 isoforms by siRNA prevents the ER stress-associated decrease of p21 in HCT116 cells. ( b ) Treatment of cells with a 1 μM doxorubicin pulse (see Methods) induces DNA damage and activates the ATM kinase, as determined using a phosphospecific serine 1981 antibody (S1981-pATM). In a and b , cell lysates were analysed by western blot analysis. ACMDD serum was used to detect endogenous p53 isoforms levels in HCT116 and A549 (see Methods). BiP was used as a positive control for UPR activation and β-actin or Hsp90α+β as a loading control. Numbers shown below the bands represent p21 or S1981-pATM quantification. Blots represent n ≥3. EV stands for empty vector and p53 FL for full-length p53 (see also Supplementary Fig. 1 ). Full size image The induction of p21 by p53 forms a cornerstone in the DNA damage response and we were interested to know how cells coordinate p21 expression when both the DNA damage and the ER stress pathways are active. Cells expressing either endogenous wild-type p53 or cells in which p53 expression was introduced were treated with thapsigargin (100 nM, 16 h) and/or with the DNA damaging drug doxorubicin (Dox; 1 μM pulse). The UPR lowered, but did not prevent, DNA damage-induced phosphorylation of ataxia telangiectasia mutated (ATM) at serine 1981 (S1981-pATM). Moreover, the UPR did not alter basal levels of S1981-pATM and did not affect the downstream pathway of ATM as determined by the ratio of phosphorylated p53 at serine 15 (S15-pp53 FL) over the total amount of p53 FL ( Fig. 1b and Supplementary Fig. 1a ). However, exposure to thapsigargin prevented the induction of p21 following genotoxic stress in A549 and HCT116 cells as well as in H1299 and Saos-2 cells expressing p53 ( Fig. 1b ). The induction of p21 in p53-expressing H1299 cells or in A549 cells following treatment with Dox was also prevented by tunicamycin (7.5 μg ml −1 for 16 h), which induces ER stress by interfering with protein glycosylation ( Supplementary Fig. 1b,2c ). Suppression of p21 enhances DNA damage-induced apoptosis The activity of p21 normally subdues p53-induced apoptosis following DNA damage and we next measured apoptosis in Dox-treated cells with, or without, activated UPR. Cells were treated with thapsigargin for 16 h (100 nM) and Dox was added for the last hour (1 μM). HCT116 cells subjected to this double treatment showed an over sixfold increase in the relative change of early apoptosis and an over threefold increase in late apoptosis, as compared with cells treated with Dox alone. The corresponding increase in early apoptosis for this double treatment was over 1.6-fold as compared with cells treated with thapsigargin alone and with no significant relative change in late apoptosis ( Fig. 2a , graph and dot plots and Supplementary Fig. 2a ). Interestingly, overexpression of exogenous p21 (0.50 μg) reversed the increase in p53-dependent early apoptosis observed following double stress, as compared with DNA damage alone ( Fig. 2b , graph and dot plots). In a similar way, the p53-dependent apoptosis in Saos-2 cells subjected to combined ER and genotoxic stress was reduced by 40% when overexpressing p21 ( Supplementary Fig. 2b ). The p53-dependent apoptosis under double stress conditions was further illustrated with a 50% reversal when p53 levels were suppressed using siRNA ( Fig. 2c ). The induction of apoptosis was accompanied by an increase in cleaved poly (ADP-ribose) polymerase (PARP) and active caspase 7 over a 16-h time course that was higher in cells undergoing double genotoxic and ER stress, as compared with either stress alone. On the contrary, expression of the ER-linked pro-apoptotic C/EBP homology protein (CHOP) was increased to a similar extent after double treatment or after thapsigargin alone. DNA damage did not prevent chemical induction of the UPR and vice versa , activation of the ATM pathway was not affected by ER stress, as indicated by induction of BiP and phosphorylation of the downstream ATM target p53 at serine 15 (S15-pp53FL), respectively ( Fig. 2d and Supplementary Fig. 2c ). Altogether, these results show that the DNA damage-induced increase in p21 expression is suppressed in cells undergoing the UPR and that this correlates with a change in the ratio of p53/47:p53 FL. The failure to induce p21 results in a lowered p53-dependent apoptotic threshold. 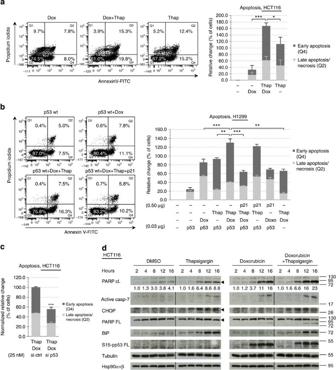Figure 2: Suppression of p21 during ER stress sensitizes cells to p53- and DNA damage-induced apoptosis. (a) HCT116 or (b) H1299 cells expressing p53- and/or p21-encoding constructs as indicated, were treated as in (Fig. 1b) and analysed for apoptosis by FACS after staining with Annexin V-FITC and propidium iodide (PI). Representative dot plots show the discrimination of viable cells (FITC−PI−, lower left Q3), early apoptotic (FITC+PI−, lower right Q4) and late apoptotic or necrotic cells (FITC+PI+, upper right quadrant Q2). Graphs show the relative change in percentage of cells in early apoptosis and late apoptosis/necrosis compared with empty vector (EV)-transfected and DMSO-treated cells, set to zero. (c) Relative effect on apoptosis after suppression of p53 expression using siRNA in HCT116 cells exposed to ER stress and DNA damage. Values were normalized with corresponding DMSO-treated cells and are compared with control siRNA (si ctrl) transfected cells, set to 100. (d) Levels of pro-apoptotic (CHOP) and apoptotic markers (cleaved PARP and active caspase-7) in HCT116 treated with 0.1% DMSO, 100 nM thapsigargin and/or 1 μM doxorubicin for the indicated times. The phosphorylation of p53 on serine 15 (S15) is ATM-dependent. BiP confirmed UPR activation. Tubulin and Hsp90α+β were used as loading controls. Numbers shown represent cleaved PARP quantification. Graphical data represent mean±s.d.,n≥3 performed in duplicates. Student’st-test compared data to the reference point or as indicated (*P<0.05; **P<0.01; ***P<0.001; see alsoSupplementary Fig. 2). Figure 2: Suppression of p21 during ER stress sensitizes cells to p53- and DNA damage-induced apoptosis. ( a ) HCT116 or ( b ) H1299 cells expressing p53- and/or p21-encoding constructs as indicated, were treated as in (Fig. 1b) and analysed for apoptosis by FACS after staining with Annexin V-FITC and propidium iodide (PI). Representative dot plots show the discrimination of viable cells (FITC − PI − , lower left Q3), early apoptotic (FITC + PI − , lower right Q4) and late apoptotic or necrotic cells (FITC + PI + , upper right quadrant Q2). Graphs show the relative change in percentage of cells in early apoptosis and late apoptosis/necrosis compared with empty vector (EV)-transfected and DMSO-treated cells, set to zero. ( c ) Relative effect on apoptosis after suppression of p53 expression using siRNA in HCT116 cells exposed to ER stress and DNA damage. Values were normalized with corresponding DMSO-treated cells and are compared with control siRNA (si ctrl) transfected cells, set to 100. ( d ) Levels of pro-apoptotic (CHOP) and apoptotic markers (cleaved PARP and active caspase-7) in HCT116 treated with 0.1% DMSO, 100 nM thapsigargin and/or 1 μM doxorubicin for the indicated times. The phosphorylation of p53 on serine 15 (S15) is ATM-dependent. BiP confirmed UPR activation. Tubulin and Hsp90α+β were used as loading controls. Numbers shown represent cleaved PARP quantification. Graphical data represent mean±s.d., n ≥3 performed in duplicates. Student’s t -test compared data to the reference point or as indicated (* P <0.05; ** P <0.01; *** P <0.001; see also Supplementary Fig. 2 ). Full size image p53/47 regulates full-length p53-induced p21 transcription We next investigated if the induction of p53/47 following activation of the UPR is responsible for the suppression of p21 expression. Increasing p53/47 levels (0.06 to 0.50 μg) in the presence of a fixed amount of p53 FL (0.50 μg) revealed a p53/47 dose-dependent reduction in endogenous p21 levels with 80% suppression at 0.50 μg. In cells undergoing ER stress, the suppression of p21 was even more impressive with an approximately 70% reduction already at 0.13 μg of p53/47 ( Fig. 3a,b ). Real-time quantitative PCR (RT–qPCR) under the same conditions showed that p53 FL alone induced an approximately 13-fold increase in p21 mRNA levels that was gradually suppressed by p53/47 with no significant difference between cells treated, or not, with thapsigargin ( Fig. 3c ). We also measured p21 promoter activity using a firefly luciferase (FLuc) reporter construct and we observed a similar progressive suppression of p53 FL activity with increasing p53/47 levels, independently if cells had been exposed, or not, to thapsigargin ( Fig. 3d ). However, the observed reduction at the p21 promoter activity and p21 mRNA levels did not reflect the nearly complete suppression of the p21 protein. Hence, these results identified p53/47 as a suppressor of p53 FL-mediated transactivation of the p21 promoter, but they do not fully explain the p53-dependent suppression of p21 protein expression during the UPR. 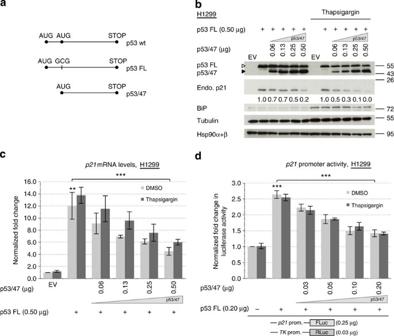Figure 3: ER stress-induced expression of p53/47 prevents activation ofp21transcription by p53 FL. (a) Schematic representation of the p53-expressing constructs used. The p53 wt construct contains coding sequence and initiation codons for both full-length p53 (p53 FL) and p53/47 and encodes both isoforms. The AUG initiation codon for p53/47 was substituted to an alanine (GCG) in the p53 FL-expressing construct. Sequence upstream of the p53/47 initiation codon (+1 to +120 nt) was deleted in the p53/47-expressing construct. (b) Endogenous p21 protein levels following expression of increased p53/47 levels in the presence of a fixed amount of p53 FL in H1299 cells treated, or not, with thapsigargin (100 nM, 16 h). Tubulin and Hsp90α+β served as loading controls. Numbers shown below bands represent p21 quantification. Immunoblots representn≥3. (c) Samples frombwere analysed in parallel for the effect of p53 isoforms expression on endogenousp21mRNA levels using RT–qPCR. Values were normalized againstactinand are presented as fold change relative to empty vector (EV)-transfected and DMSO-treated cells, set to 1 (mean±s.d.,n≥3 performed in duplicates). (d)p21promoter activity. Reporter constructsp21promoter-FLuc (firefly luciferase) andTK(thymidine kinase) promoter-RLuc (Renillaluciferase) were co-transfected and dual luciferase assay was performed. Activity of FLuc was normalized to that of RLuc. Values are shown as fold change in luciferase activity compared with p53 non-transfected and DMSO-treated cells, set to 1 (mean±s.d.,n≥3 performed in triplicates). Incandd, Student’st-test was performed to compare data to the reference point or as indicated (**P<0.01; ***P<0.001). Figure 3: ER stress-induced expression of p53/47 prevents activation of p21 transcription by p53 FL. ( a ) Schematic representation of the p53-expressing constructs used. The p53 wt construct contains coding sequence and initiation codons for both full-length p53 (p53 FL) and p53/47 and encodes both isoforms. The AUG initiation codon for p53/47 was substituted to an alanine (GCG) in the p53 FL-expressing construct. Sequence upstream of the p53/47 initiation codon (+1 to +120 nt) was deleted in the p53/47-expressing construct. ( b ) Endogenous p21 protein levels following expression of increased p53/47 levels in the presence of a fixed amount of p53 FL in H1299 cells treated, or not, with thapsigargin (100 nM, 16 h). Tubulin and Hsp90α+β served as loading controls. Numbers shown below bands represent p21 quantification. Immunoblots represent n ≥3. ( c ) Samples from b were analysed in parallel for the effect of p53 isoforms expression on endogenous p21 mRNA levels using RT–qPCR. Values were normalized against actin and are presented as fold change relative to empty vector (EV)-transfected and DMSO-treated cells, set to 1 (mean±s.d., n ≥3 performed in duplicates). ( d ) p21 promoter activity. Reporter constructs p21 promoter-FLuc (firefly luciferase) and TK (thymidine kinase) promoter-RLuc ( Renilla luciferase) were co-transfected and dual luciferase assay was performed. Activity of FLuc was normalized to that of RLuc. Values are shown as fold change in luciferase activity compared with p53 non-transfected and DMSO-treated cells, set to 1 (mean±s.d., n ≥3 performed in triplicates). In c and d , Student’s t -test was performed to compare data to the reference point or as indicated (** P <0.01; *** P <0.001). Full size image Suppression of p21 expression by p53 isoforms To identify at which additional level p53/47 might repress p21 expression, we instead increased the levels of p53 FL (0.06–0.50 μg) in the presence of a fixed amount of p53/47 (0.50 μg). This resulted in a dose-dependent elevation of p21 protein levels with an approximately sixfold induction at 0.50 μg. However, in the presence of thapsigargin, although p53 FL still induced p21 mRNA levels, induction of p21 protein expression was abrogated by nearly 50%, as compared with non-treated cells. In fact, the induction of p21 mRNA levels by 0.50 μg of p53 FL was significantly higher during ER stress ( Fig. 4a,b ). Notably, p53/47 expression alone resulted in a slight but significant increase in endogenous p21 mRNA and protein levels as well as p21 promoter-FLuc activity, in line with a previous report showing that p53/47 has a weak positive effect on the endogenous p21 promoter in the absence of full-length p53 (ref. 16; Fig. 4a–c and Supplementary Fig. 3a ). Hence, even though p53/47 by itself can induce a limited p21 expression, it is an effective inhibitor of p53 FL activity towards p21 promoter. Previous studies have shown that p53/47 forms tetramers more easily as compared with p53 FL during the UPR and we could now also observe an approximately tenfold stronger affinity of p53/47, as compared with p53 FL, towards the p21 promoter as estimated from chromatin immunoprecipitation (ChIP) assays ( Supplementary Fig. 3b ) [23] . Plotting the p53 FL dose-dependent ratio of p21 protein over p21 mRNA illustrates how an increase in p21 mRNA levels does not translate into p21 protein expression in the presence of p53/47 and during ER stress ( Fig. 4d ). 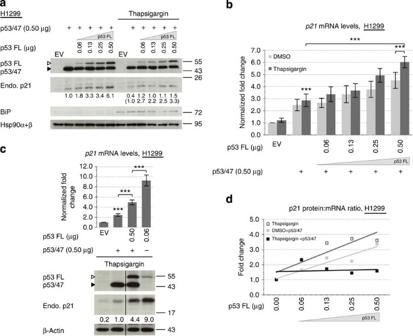Figure 4: p53/47 controls expression of p21 at transcriptional and post-transcriptional levels. (a) Effect of p53/47 on p53 FL-dependent induction of p21 protein levels during ER stress conditions. H1299 cells were transfected with a fixed amount of p53/47 and increasing p53 FL and treated with thapsigargin or DMSO, followed by immunoblotting. (b) Samples fromawere analysed by RT–qPCR to estimatep21mRNA levels. Values were normalized againstactinand are presented in fold change relative to empty vector (EV)-transfected and DMSO-treated cells, set to 1 (mean±s.d.,n≥3 performed in duplicates). (c)p21mRNA and protein levels were assessed in the presence of p53 isoforms, as indicated, during thapsigargin treatment. mRNA values are relative to EV-transfected cells, set to 1 (mean±s.d.,n≥3, in duplicates). Inbandc, Student’st-test was performed to compare data to the reference point or as indicated (***P<0.001). Inaandc, Hsp90α+β or β-actin served as loading controls. Numbers shown below the bands represent p21 quantification. Blots representn≥3. (d) p53 FL dose-dependent ratio of densitometric values of p21 protein levels on normalized fold change inp21mRNA levels froma–cis shown in graphic form. Linear regression curves are displayed (see alsoSupplementary Fig. 3). Figure 4: p53/47 controls expression of p21 at transcriptional and post-transcriptional levels. ( a ) Effect of p53/47 on p53 FL-dependent induction of p21 protein levels during ER stress conditions. H1299 cells were transfected with a fixed amount of p53/47 and increasing p53 FL and treated with thapsigargin or DMSO, followed by immunoblotting. ( b ) Samples from a were analysed by RT–qPCR to estimate p21 mRNA levels. Values were normalized against actin and are presented in fold change relative to empty vector (EV)-transfected and DMSO-treated cells, set to 1 (mean±s.d., n ≥3 performed in duplicates). ( c ) p21 mRNA and protein levels were assessed in the presence of p53 isoforms, as indicated, during thapsigargin treatment. mRNA values are relative to EV-transfected cells, set to 1 (mean±s.d., n ≥3, in duplicates). In b and c , Student’s t -test was performed to compare data to the reference point or as indicated (*** P <0.001). In a and c , Hsp90α+β or β-actin served as loading controls. Numbers shown below the bands represent p21 quantification. Blots represent n ≥3. ( d ) p53 FL dose-dependent ratio of densitometric values of p21 protein levels on normalized fold change in p21 mRNA levels from a – c is shown in graphic form. Linear regression curves are displayed (see also Supplementary Fig. 3 ). Full size image p53 isoforms control p21 mRNA translation To visualize the post-transcriptional effect of p53/47 on p21, we expressed a constant amount (0.50 μg) of an exogenous p21-coding sequence (CDS) under control of the cytomegalovirus (CMV) promoter while increasing the levels of p53/47 (0.13–1.00 μg) in ER-stressed H1299 cells. This resulted in a progressive (up to 80%) reduction in ectopic p21 protein levels without affecting the levels of exogenous p21 mRNA ( Fig. 5a ). The decrease in p21 levels was also observed using an anti-FLAG antibody towards an N-terminally 3X FLAG-tagged p21 and was more pronounced in cells treated with thapsigargin ( Fig. 5b ). A similar reduction in exogenous p21 protein levels by p53/47 during the UPR could also be observed in HCT116, U2OS and MLS-1765 cells ( Supplementary Fig. 4 ). 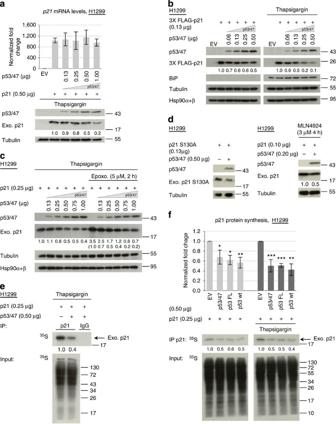Figure 5: p53/47 and p53 FL inhibit p21 protein synthesis. (a) Effect of increasing amounts of p53/47 on p21 mRNA and protein levels in H1299 cells expressing ectopic p21 (0.50 μg cDNA). RT–qPCR using primers within thep21-coding sequence detected both endogenous and exogenousp21mRNAs (the latter is restricted to the coding sequence). Values were normalized againstactinand are relative to endogenous levels in empty vector (EV)-transfected cells, set to 1 (mean±s.d.,n≥3, performed in duplicates). (b) The inhibition of ectopic p21 protein expression by increasing amounts of p53/47 was verified under normal and ER stress conditions using an N-terminally 3X FLAG-tagged p21 and anti-FLAG antibody. (c) Effect on p21 protein expression using increasing p53/47 levels, while inhibiting proteasomal degradation with 5 μM epoxomicin (epoxo.) during the last 2 h of thapsigargin treatment. (d) p53/47 suppresses expression of the p21 S130A mutant that is not targeted for ubiquitin-dependent proteasomal degradation by the SCFSKP2(SKP1/CUL-1/SKP2) complex and of wild-type p21 in cells treated with the MLN4924 molecule (3 μM for 4 h) that inactivates the SCFSKP2complex. Ina–d, Hsp90α+β and/or tubulin served as control for equal loading. Numbers shown below the bands represent p21 quantification. Blots representn≥3. (e)De novop21 protein synthesis. Cells expressing p21 in the presence or absence of p53/47 under thapsigargin treatment were metabolically pulse labelled with35S-methionine (45 μCi ml−1) for 30 min in the presence of proteasome inhibitor. Cell extracts were immunoprecipitated (IP) with p21 or non-specific IgG antibody. Levels of IP radiolabelled protein were assessed by autoradiography and quantified. Input samples served as control for equal incorporation of35S-methionine into cellular proteins. Autoradiograph shown is representative ofn≥3. (f) Cells were transfected with p21 together with p53/47, p53 FL or p53 wt constructs and treated, or not, with thapsigargin. Samples were analysed forde novop21 protein synthesis as ine. Graph shows values relative to the corresponding EV-transfected cells, set to 1 (mean±s.d.,n≥3). Student’st-test compared data to the reference point (*P<0.05; **P<0.01; ***P<0.001). A representative autoradiograph is shown below (see alsoSupplementary Fig. 4). Figure 5: p53/47 and p53 FL inhibit p21 protein synthesis. ( a ) Effect of increasing amounts of p53/47 on p21 mRNA and protein levels in H1299 cells expressing ectopic p21 (0.50 μg cDNA). RT–qPCR using primers within the p21 -coding sequence detected both endogenous and exogenous p21 mRNAs (the latter is restricted to the coding sequence). Values were normalized against actin and are relative to endogenous levels in empty vector (EV)-transfected cells, set to 1 (mean±s.d., n ≥3, performed in duplicates). ( b ) The inhibition of ectopic p21 protein expression by increasing amounts of p53/47 was verified under normal and ER stress conditions using an N-terminally 3X FLAG-tagged p21 and anti-FLAG antibody. ( c ) Effect on p21 protein expression using increasing p53/47 levels, while inhibiting proteasomal degradation with 5 μM epoxomicin (epoxo.) during the last 2 h of thapsigargin treatment. ( d ) p53/47 suppresses expression of the p21 S130A mutant that is not targeted for ubiquitin-dependent proteasomal degradation by the SCF SKP2 (SKP1/CUL-1/SKP2) complex and of wild-type p21 in cells treated with the MLN4924 molecule (3 μM for 4 h) that inactivates the SCF SKP2 complex. In a – d , Hsp90α+β and/or tubulin served as control for equal loading. Numbers shown below the bands represent p21 quantification. Blots represent n ≥3. ( e ) De novo p21 protein synthesis. Cells expressing p21 in the presence or absence of p53/47 under thapsigargin treatment were metabolically pulse labelled with 35 S-methionine (45 μCi ml −1 ) for 30 min in the presence of proteasome inhibitor. Cell extracts were immunoprecipitated (IP) with p21 or non-specific IgG antibody. Levels of IP radiolabelled protein were assessed by autoradiography and quantified. Input samples served as control for equal incorporation of 35 S-methionine into cellular proteins. Autoradiograph shown is representative of n ≥3. ( f ) Cells were transfected with p21 together with p53/47, p53 FL or p53 wt constructs and treated, or not, with thapsigargin. Samples were analysed for de novo p21 protein synthesis as in e . Graph shows values relative to the corresponding EV-transfected cells, set to 1 (mean±s.d., n ≥3). Student’s t -test compared data to the reference point (* P <0.05; ** P <0.01; *** P <0.001). A representative autoradiograph is shown below (see also Supplementary Fig. 4 ). Full size image We next addressed if the post-transcriptional regulation of p21 expression by p53/47 relates to p21 stability or synthesis. Expressing a fixed amount of exogenous p21 (0.25 μg) in H1299 cells treated with 5 μM of the proteasome inhibitor epoxomicin for 2 h under ER stress resulted in a 3.5-fold elevation in p21 levels. However, increasing the amount of p53/47 (0.13–1.00 μg) resulted in a similar reduction in p21 expression in cells treated, or not, with epoxomicin ( Fig. 5c ). Either mutating serine 130 of p21 to alanine (p21 S130A) to prevent ubiquitin-dependent proteasomal degradation of p21 by the SCF SKP2 (SKP1/CUL-1/SKP2) complex [57] , [58] or treating cells with the Nedd8 ligase inhibitor MLN4924 to inhibit SCF SKP2 activity [59] , had little effect on p53/47-mediated inhibition of p21 ( Fig. 5d ). When we instead tested p53/47’s effect on p21 mRNA translation using 35 S-methionine metabolic pulse labelling in the presence of proteasome inhibitor, we observed a 60% reduction in the rate of p21 de novo synthesis ( Fig. 5e ). As the ectopic p21 mRNA levels are not changed by p53/47, these observations demonstrate that p53/47 represses p21 mRNA translation. When we compared the repression of de novo p21 protein synthesis by p53 FL, p53/47 or a combination of the two isoforms, we made a further surprising observation in that both isoforms suppressed p21 mRNA translation to a similar extent ( Fig. 5f ). p53 targets the p21 mRNA CDS to suppress its translation To assess if suppression of p21 mRNA translation requires p53 transcriptional activity, we introduced mutations in p53/47, p53 FL and p53 wt constructs to prevent their specific DNA-binding capacity. The conformation mutant R175H and the DNA contact mutants R273H and R248W [60] were expressed at similar levels as their wild-type counterparts but had no effect on exogenous, or endogenous, p21 protein levels, indicating that p53-dependent inhibition of p21 protein synthesis occurs from transcriptionally active p53 ( Fig. 6a and Supplementary Fig. 5 ). 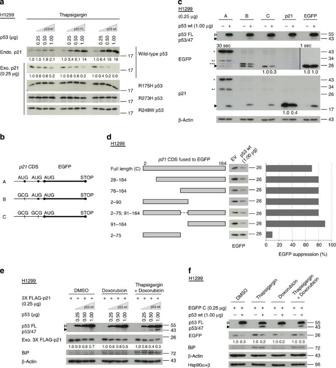Figure 6: Suppression ofp21mRNA translation by active p53 isoforms is mediated by thep21mRNA-coding sequence (CDS). (a) H1299 cells expressing wild-type p53/47, p53 FL, p53 wt constructs, or the inactive mutants R175H (conformation-DNA binding mutant), R273H or R248W (contact site-DNA binding mutants). Empty vector or CMV promoter-driven p21 was co-expressed and cells were treated with thapsigargin (100 nM, 16 h). The effect on endogenous (endo. p21) and exogenous (exo. p21) p21 protein levels was assessed by western blot analysis. (b) Schematic representation of thep21mRNA-CDS fused to the enhanced green fluorescent protein (EGFP) reporter constructs. Thep21CDS with no stop codon was subcloned in front of theEGFPopen reading frame (A). The first (B) or both (C) in-frame p21 AUGs were substituted with alanine (GCG). (c) Effect of p53 wt on the expression of thep21mRNA CDS-EGFPreporter constructs described inb, of p21 or EGFP alone, as assessed by western blot. Arrow heads designate EGFP and p21 proteins, whereas asterisks indicate p21-EGFP fusion products. Different exposure times are indicated above. (d) Deletions within thep21mRNA CDS (construct C) are schematically depicted (left). Numbers indicate included codons. Effect of p53 wt on the EGFP expression from these constructs is shown (middle) and corresponding quantification is reported as the percentage of EGFP suppression (right graph). (e) Effect of p53 wt on the expression of exogenous 3X FLAG-tagged p21 under different conditions (DMSO, doxorubicin or doxorubicin plus thapsigargin treatment, all 100 nM, 16 h) as estimated by immunoblotting. (f) Similar toe, but using thep21mRNA CDS-EGFPreporter construct. Ina–f, numbers shown below the bands represent quantification of corresponding proteins. Blots representn≥3 (see alsoSupplementary Fig. 5). Figure 6: Suppression of p21 mRNA translation by active p53 isoforms is mediated by the p21 mRNA-coding sequence (CDS). ( a ) H1299 cells expressing wild-type p53/47, p53 FL, p53 wt constructs, or the inactive mutants R175H (conformation-DNA binding mutant), R273H or R248W (contact site-DNA binding mutants). Empty vector or CMV promoter-driven p21 was co-expressed and cells were treated with thapsigargin (100 nM, 16 h). The effect on endogenous (endo. p21) and exogenous (exo. p21) p21 protein levels was assessed by western blot analysis. ( b ) Schematic representation of the p21 mRNA-CDS fused to the enhanced green fluorescent protein (EGFP) reporter constructs. The p21 CDS with no stop codon was subcloned in front of the EGFP open reading frame (A). The first (B) or both (C) in-frame p21 AUGs were substituted with alanine (GCG). ( c ) Effect of p53 wt on the expression of the p21 mRNA CDS- EGFP reporter constructs described in b , of p21 or EGFP alone, as assessed by western blot. Arrow heads designate EGFP and p21 proteins, whereas asterisks indicate p21-EGFP fusion products. Different exposure times are indicated above. ( d ) Deletions within the p21 mRNA CDS (construct C) are schematically depicted (left). Numbers indicate included codons. Effect of p53 wt on the EGFP expression from these constructs is shown (middle) and corresponding quantification is reported as the percentage of EGFP suppression (right graph). ( e ) Effect of p53 wt on the expression of exogenous 3X FLAG-tagged p21 under different conditions (DMSO, doxorubicin or doxorubicin plus thapsigargin treatment, all 100 nM, 16 h) as estimated by immunoblotting. ( f ) Similar to e , but using the p21 mRNA CDS- EGFP reporter construct. In a – f , numbers shown below the bands represent quantification of corresponding proteins. Blots represent n ≥3 (see also Supplementary Fig. 5 ). Full size image Insertion of a p21 mRNA CDS in which the in frame AUG codons had been substituted with alanines, in front of the EGFP open reading frame resulted in a 70% reduction in enhanced green fluorescent protein (EGFP) levels in the presence of p53 wt, whereas EGFP expressed from a vector carrying no p21 mRNA remained unchanged ( Fig. 6b,c ). These reporter constructs confirmed that the CDS of the p21 mRNA is sufficient and necessary for the effect of p53 isoforms on mRNA translation, with no requirement for p21 protein synthesis. A series of deletions was generated within the p21 mRNA CDS and two regions in the central (codons 76–90) and in the 3′ (91 to 164) were identified to mediate p53-dependent inhibition of translation ( Fig. 6d ). This indicates that the p53 response element spans a large bi-part region of the p21 mRNA, making it unlikely that the target of p53 activity to control p21 synthesis is via a single microRNA (miRNA), and instead points towards a structure-dependent protein–RNA interaction. Furthermore, the two p53-induced miRNAs [61] described to target the p21 mRNA CDS (miR-194 and 15a) interact within the first 73 codons. We could observe an inhibition of synthesis from 3X FLAG-tagged p21 mRNA and from the p21 mRNA-EGFP constructs by p53 wt in the presence of dimethyl sulfoxide (DMSO), Dox or Dox plus thapsigargin ( Fig. 6e,f ). Hence, the capacity of p53 to control p21 mRNA translation does not appear to be strict condition dependent. p21 impairs p53/47-induced G2 arrest during ER stress We next set out to investigate how the suppression of p21 relates to p53-induced G2 arrest following ER stress. H1299 cells overexpressing the p53/47 isoform (0.50 μg) under thapsigargin treatment were transfected with increasing amounts of p21 and the cell cycle distribution in non-synchronized cells was determined by fluorescence-activated cell sorting (FACS) analysis. A progressive reduction in p53/47-induced G2 arrest up to 20% was observed while at the same time the number of cells in G1 increased by approximately 7% ( Fig. 7a and Supplementary Fig. 6 ). Increasing amounts of p21 in MLS-1765 cells [23] expressing wild-type p53 also resulted in a gradual decrease (20%) in ER stress-induced G2 arrest, while at the same time the population of cells in G1 increased (15%; Fig. 7b ). Similarly, two additional cell lines that respond with G2 arrest following ER stress, HCT116 and A549, each showed an approximately 5% induction in G1 and a nearly 15% decrease in p53/47-dependent G2 arrest following introduction of p21 ( Fig. 7c ). When we instead knocked down endogenous p21 using siRNA we observed an approximately 15% increase in p53/47-dependent G2 arrest and a concomitant 5% reduction in the number of cells in G1 following treatment with thapsigargin ( Fig. 7d ). We also observed that a p53/47 dose-dependent reduction in ectopic p21 protein levels resulted in similar 15% increase and 5% decrease in G2- and G1-arrested cells, respectively ( Fig. 7e ). Taken together, these results reveal that p21 prevents p53/47-dependent G2/M arrest during the UPR. 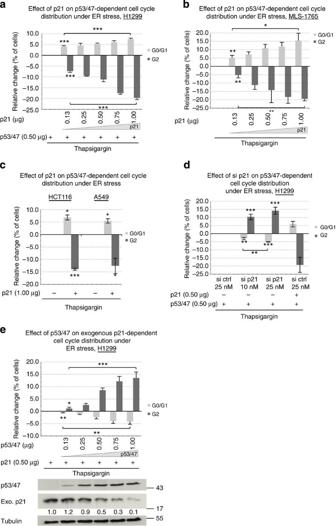Figure 7: p21 suppression is required for ER stress-induced G2 arrest. (a–e) Cell cycle distribution. Cells were fixed and stained with PI for DNA content analysis by FACS. p21-dependent effects on cell cycle progression in (a) p53/47-overexpressing H1299 cells or p53-positive (b) MLS-1765 and (c) HCT116 and A549 cells, treated with thapsigargin. Results are presented as the relative change in percentage of cells arrested in G0/G1 and G2 compared with cells where no p21 was overexpressed, set to zero. (d) H1299 cells overexpressing p53/47 in combination with siRNA specific top21(si p21), non-targeting control siRNA (si ctrl) or p21-encoding vector. Values show the relative change in percentage of cells arrested in G0/G1 and G2 compared with p53/47 and si ctrl-transfected cells, set to zero. (e) A fixed amount of ectopic p21 was expressed together with increasing p53/47 levels. Results are presented in relative change as compared with p53/47 non-transfected cells, set to zero. Corresponding levels of p21 and p53/47 proteins were assessed by western blot and are shown below (representative ofn≥3). Numbers represent quantification of p21 expression. Ina–e, graphs represent mean±s.d. ofn≥3, performed in triplicates. Student’st-test compared data to the reference point or as indicated (*P<0.05; **P<0.01; ***P<0.001; see alsoSupplementary Fig. 6). Figure 7: p21 suppression is required for ER stress-induced G2 arrest. ( a – e ) Cell cycle distribution. Cells were fixed and stained with PI for DNA content analysis by FACS. p21-dependent effects on cell cycle progression in ( a ) p53/47-overexpressing H1299 cells or p53-positive ( b ) MLS-1765 and ( c ) HCT116 and A549 cells, treated with thapsigargin. Results are presented as the relative change in percentage of cells arrested in G0/G1 and G2 compared with cells where no p21 was overexpressed, set to zero. ( d ) H1299 cells overexpressing p53/47 in combination with siRNA specific to p21 (si p21), non-targeting control siRNA (si ctrl) or p21-encoding vector. Values show the relative change in percentage of cells arrested in G0/G1 and G2 compared with p53/47 and si ctrl-transfected cells, set to zero. ( e ) A fixed amount of ectopic p21 was expressed together with increasing p53/47 levels. Results are presented in relative change as compared with p53/47 non-transfected cells, set to zero. Corresponding levels of p21 and p53/47 proteins were assessed by western blot and are shown below (representative of n ≥3). Numbers represent quantification of p21 expression. In a – e , graphs represent mean±s.d. of n ≥3, performed in triplicates. Student’s t -test compared data to the reference point or as indicated (* P <0.05; ** P <0.01; *** P <0.001; see also Supplementary Fig. 6 ). Full size image p21 controls 14-3-3σ protein stability 14-3-3σ is required for p53/47-induced G2 arrest and we investigated if p21 is linked to 14-3-3σ activity. Increasing p21 levels during the UPR resulted in a dose-dependent reduction in 14-3-3σ, whereas siRNA-mediated downregulation of endogenous p21 resulted in a concordant increase in 14-3-3σ levels ( Fig. 8a and Supplementary Fig. 7a ). To test if this effect of p21 could be indirect via G1 cell cycle arrest, we instead introduced increasing levels of the cyclin D/CDK4-6 inhibitor p16 INK4A . However, p16 did not alter 14-3-3σ protein levels, indicating that suppression of 14-3-3σ relates to a novel and particular function of p21 and not to G1 arrest per se ( Fig. 8b ). We also observed a comparable downregulation of 14-3-3σ by p21 in HCT116, MLS-1765 and U2OS, all of which express detectable levels of 14-3-3σ ( Fig. 8c ). In addition, p53/47-mediated inhibition of p21 levels resulted in a concomitant increase in endogenous 14-3-3σ levels ( Fig. 8d ). Elevation of p53/47 in MLS-1765 cells resulted in a similar 30% decrease in exogenous p21 and in a 2.4-fold increase in endogenous 14-3-3σ, showing that p53/47-mediated suppression of p21 is sufficient to induce 14-3-3σ ( Supplementary Fig. 7b ). Furthermore, p21-null HCT116 cells (HCT116 p21 −/− ) showed an elevated expression of 14-3-3σ, as compared with HCT116 (p21 +/+ ) cells, that was reduced after reintroduction of ectopic p21 (0.25 μg; Fig. 8e ). 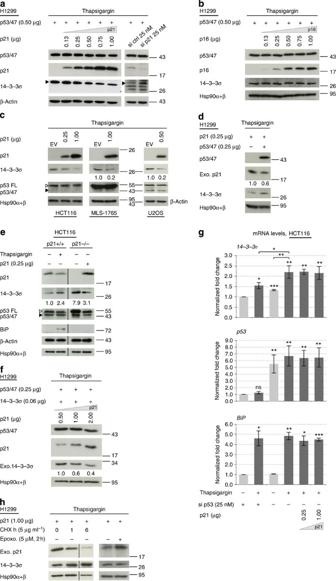Figure 8: p21 affects 14-3-3σ protein stability. (a) Immunoblot showing the effect of p21 on 14-3-3 sigma (14-3-3σ) protein expression. H1299 cells overexpressing p53/47 under thapsigargin treatment were transfected with increasing amounts of p21; or endogenous p21 levels were suppressed usingp21siRNA (si p21). (b) Similar toa(left panel), but increasing the amount of the cyclin D/CDK4-6 inhibitor p16INK4ainstead of p21. (c) Downregulation of 14-3-3σ by increased p21 levels in HCT116, MLS-1765 and U2OS cells. (d) p53/47-mediated suppression of ectopic p21 expression increases 14-3-3σ levels in H1299 cells. (e) Expression of 14-3-3σ and p53 isoforms in HCT116 or HCT116 p21−/−cells following ER stress or reintroduction of p21. (f) Suppression of exogenous 14-3-3σ by p21. H1299 cells expressed a fixed amount of p53/47 and 14-3-3σ together with increasing levels of p21. (g) HCT116 cells transfected with p53-specific, or control, siRNA together with empty vector (EV) or increasing amount of p21 were treated, or not, with thapsigargin. RT–qPCR was performed to measure14-3-3σ,p53andBiPmRNA levels.GAPDH-normalized values are presented in fold change relative to DMSO-treated and si p53-transfected cells, which were assigned a value of 1 (mean±s.d.,n≥3, in duplicates). Student’st-test was carried out by comparing data to the reference point (*P<0.05; **P<0.01; ***P<0.001). (h) H1299 cells expressing ectopic p21 were treated with the protein synthesis inhibitor cycloheximide (CHX) at 5 μg ml−1for 0–6 h or with the proteasome inhibitor epoxomicin (epoxo.) at 5 μM for 2 h. p21 and 14-3-3σ protein levels were assessed by western blot. Ina–f,h, β-actin and Hsp90α+β served as loading controls and numbers shown below the bands represent quantification of corresponding proteins. Blots are representative ofn≥3 (see alsoSupplementary Fig. 7). Figure 8: p21 affects 14-3-3σ protein stability. ( a ) Immunoblot showing the effect of p21 on 14-3-3 sigma (14-3-3σ) protein expression. H1299 cells overexpressing p53/47 under thapsigargin treatment were transfected with increasing amounts of p21; or endogenous p21 levels were suppressed using p21 siRNA (si p21). ( b ) Similar to a (left panel), but increasing the amount of the cyclin D/CDK4-6 inhibitor p16 INK4a instead of p21. ( c ) Downregulation of 14-3-3σ by increased p21 levels in HCT116, MLS-1765 and U2OS cells. ( d ) p53/47-mediated suppression of ectopic p21 expression increases 14-3-3σ levels in H1299 cells. ( e ) Expression of 14-3-3σ and p53 isoforms in HCT116 or HCT116 p21 −/− cells following ER stress or reintroduction of p21. ( f ) Suppression of exogenous 14-3-3σ by p21. H1299 cells expressed a fixed amount of p53/47 and 14-3-3σ together with increasing levels of p21. ( g ) HCT116 cells transfected with p53-specific, or control, siRNA together with empty vector (EV) or increasing amount of p21 were treated, or not, with thapsigargin. RT–qPCR was performed to measure 14-3-3σ , p53 and BiP mRNA levels. GAPDH -normalized values are presented in fold change relative to DMSO-treated and si p53-transfected cells, which were assigned a value of 1 (mean±s.d., n ≥3, in duplicates). Student’s t -test was carried out by comparing data to the reference point (* P <0.05; ** P <0.01; *** P <0.001). ( h ) H1299 cells expressing ectopic p21 were treated with the protein synthesis inhibitor cycloheximide (CHX) at 5 μg ml −1 for 0–6 h or with the proteasome inhibitor epoxomicin (epoxo.) at 5 μM for 2 h. p21 and 14-3-3σ protein levels were assessed by western blot. In a – f , h , β-actin and Hsp90α+β served as loading controls and numbers shown below the bands represent quantification of corresponding proteins. Blots are representative of n ≥3 (see also Supplementary Fig. 7 ). Full size image We next sought to understand at what level p21 controls 14-3-3σ expression. Increasing the amount of p21 caused a dose-dependent reduction in 14-3-3σ expressed from the CMV promoter during ER stress, pointing towards a post-transcriptional mode of regulation ( Fig. 8f and Supplementary Fig. 7c ). Furthermore, treatment of HCT116 cells with thapsigargin triggered an increase in 14-3-3σ mRNA levels that was not affected by p21, showing that the downregulation of 14-3-3σ does not result from decreased mRNA levels. Suppression of p53 using siRNA resulted in a significant, but not complete, decrease in ER stress-dependent induction of 14-3-3σ mRNA levels ( Fig. 8g ). When we treated cells with the protein synthesis inhibitor cycloheximide, we observed a progressive loss of ectopic p21 expression over 6 h, as expected, while at the same time 14-3-3σ levels increased, indicative of a higher turnover rate of p21 as compared with 14-3-3σ and an inverse correlation between p21 and 14-3-3σ expression. On the contrary, treatment with the proteasome inhibitor epoxomicin resulted in a stabilization of p21 that did not correlate with a reduction in 14-3-3σ ( Fig. 8h ). Altogether, these results indicate that p21 governs the stability of 14-3-3σ. p21 controls COP1-dependent stability of 14-3-3σ COP1 is an E3 ubiquitin ligase that targets 14-3-3σ for proteasomal degradation [35] and we confirmed that COP1 expression inversely correlates with 14-3-3σ protein levels in different cell lines that express detectable levels of 14-3-3σ ( Fig. 9a ). In order to determine if COP1 plays a role in the downregulation of 14-3-3σ by p21, we assessed the effect of p21 on exogenous 14-3-3σ (0.06 μg) while modulating COP1 expression. Knocking down COP1 resulted in a significantly reduced suppression of 14-3-3σ by p21. On the other hand, overexpression of a small amount (0.06 μg) of COP1 instead enhanced the negative effect of p21 on 14-3-3σ from 40% to approximately 80% ( Fig. 9b,c ). These results implicate COP1 as a mediator of p21-induced decrease in 14-3-3σ levels during ER stress. However, we did not observe any significant effect on COP1 expression by p21 in H1299, HCT116 or MCF-7 cells, indicating that p21 could act by targeting COP1 activity towards 14-3-3σ ( Fig. 9c,d ). In line with this notion, the levels of the COP1 substrate JUN were not affected in a p21-dependent manner, although siRNA against COP1 stabilized JUN by 2.2-fold ( Fig. 9e ). 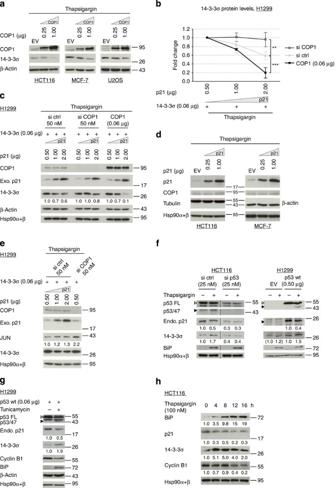Figure 9: COP1 activity is required for p21-dependent suppression of 14-3-3σ expression. (a) COP1-mediated downregulation of 14-3-3σ in cell lines expressing endogenous p53. (b) Effect of p21 on 14-3-3σ while modulating COP1 levels. H1299 cells overexpressing 14-3-3σ (0.06 μg) together with increasing amounts of p21 were co-transfected with non-targeting siRNA (si ctrl), siRNA specific toCOP1(si COP1) or low amount of COP1 cDNA. The graph displays p21 dose-dependent densitometric values of 14-3-3σ protein levels presented in fold change relative to 0.50 μg p21-transfected cells, set to 1 (mean±s.d.,n≥3). Student’st-test compared data as indicated (**P<0.01; ***P<0.001). One representative immunoblot is shown inc. (d) COP1 protein expression in HCT116 and MCF-7 p53-positive cells transfected with empty vector (EV) or increasing amount of p21. (e) Effect of p21 on the COP1 substrate JUN. H1299 cells expressing 14-3-3σ (0.06 μg) and increasing amounts of p21 in the presence of si ctrl or si COP1. (f) Suppression of p53 prevents ER stress-mediated regulation of 14-3-3σ expression. (g) H1299 cells expressing p53 wt were treated with DMSO or the ER stressor tunicamycin (7.5 μg ml−1for 16 h) and the effect on p21, 14-3-3σ and cyclin B1 expression was estimated by western blot. (h) HCT116 cells were treated with thapsigargin (100 nM) for the indicated time points and the reduction in cyclin B1 expression is indicative of p53-mediated G2 arrest. Ina–h, numbers shown below the bands indicate quantification of corresponding proteins and immunoblots representn≥3. Inf, ACMDD serum was used to detect endogenous p53 isoforms levels in HCT116 (see alsoSupplementary Fig. 8). Figure 9: COP1 activity is required for p21-dependent suppression of 14-3-3σ expression. ( a ) COP1-mediated downregulation of 14-3-3σ in cell lines expressing endogenous p53. ( b ) Effect of p21 on 14-3-3σ while modulating COP1 levels. H1299 cells overexpressing 14-3-3σ (0.06 μg) together with increasing amounts of p21 were co-transfected with non-targeting siRNA (si ctrl), siRNA specific to COP1 (si COP1) or low amount of COP1 cDNA. The graph displays p21 dose-dependent densitometric values of 14-3-3σ protein levels presented in fold change relative to 0.50 μg p21-transfected cells, set to 1 (mean±s.d., n ≥3). Student’s t -test compared data as indicated (** P <0.01; *** P <0.001). One representative immunoblot is shown in c . ( d ) COP1 protein expression in HCT116 and MCF-7 p53-positive cells transfected with empty vector (EV) or increasing amount of p21. ( e ) Effect of p21 on the COP1 substrate JUN. H1299 cells expressing 14-3-3σ (0.06 μg) and increasing amounts of p21 in the presence of si ctrl or si COP1. ( f ) Suppression of p53 prevents ER stress-mediated regulation of 14-3-3σ expression. ( g ) H1299 cells expressing p53 wt were treated with DMSO or the ER stressor tunicamycin (7.5 μg ml −1 for 16 h) and the effect on p21, 14-3-3σ and cyclin B1 expression was estimated by western blot. ( h ) HCT116 cells were treated with thapsigargin (100 nM) for the indicated time points and the reduction in cyclin B1 expression is indicative of p53-mediated G2 arrest. In a – h , numbers shown below the bands indicate quantification of corresponding proteins and immunoblots represent n ≥3. In f , ACMDD serum was used to detect endogenous p53 isoforms levels in HCT116 (see also Supplementary Fig. 8 ). Full size image To further elucidate the different steps of ER stress-dependent regulation of G2 arrest, we induced the UPR in HCT116 cells. This resulted in a 50% reduction in p21 levels and an approximately 1.7-fold increase in 14-3-3σ levels that were prevented using siRNA against p53. Concordantly, in the p53-null H1299 cells, p21 levels remained largely unchanged after UPR activation, whereas in the presence of p53 wt, the UPR caused a 60% reduction in p21 levels. The week induction of 14-3-3σ observed in H1299 following ER stress alone was significantly enhanced in the presence of p53 during the UPR ( Fig. 9f ). Similar results were obtained in H1299 cells expressing p53 wt after tunicamycin-induced ER stress ( Fig. 9g ). Finally, when we looked at the kinetics of ER stress on the expression of p21 and 14-3-3σ in HCT116 cells, we observed that when the levels of BiP started to increase during the early UPR (4 h), the expression of p21 was reduced while at the same time 14-3-3σ was increased. Later, at 12 h, the levels of cyclin B1 were reduced by more than 50%, indicative of the G2 arrest [62] ( Fig. 9h ). The suppression of ectopic p21 expression in HCT116 cells was also found to correspond to the level of the active UPR ( Supplementary Fig. 8a ). A similar reduction in cyclin B1 was observed using tunicamycin for 16 h ( Fig. 9g ). These results demonstrate that COP1 activity is required for p21-mediated regulation of 14-3-3σ. This regulation of 14-3-3σ by p21 following ER stress is independent of ATM activity ( Supplementary Fig. 8b ). The data also indicate that UPR activation is sufficient to suppress p21 in a p53-dependent manner and at the same time increase 14-3-3σ levels and trigger G2 arrest. We have studied how cells synchronize the expression and activity of p53 downstream target genes during conditions of an activated UPR and its implications for the DNA damage response. The study demonstrates a novel p53 pathway during the UPR that suppresses p21 expression in order to stabilize 14-3-3σ, induce G2 cell cycle arrest and facilitate ER damage repair. The UPR is dominant and prevents the induction of p21 following DNA damage, causing an increase in p53-mediated genotoxic-induced apoptosis. The physiological triggers of ER stress are conditions of low nutrients and/or oxygen, or pathophysiological conditions with defects in protein folding or with high protein expression levels. All are conditions that can be expected to occur in tumours. The UPR follows upon ER stress and aims at restoring the balance between newly synthesized and mature proteins. Apart from trying to rid the cell of misfolded proteins by promoting their ER-associated degradation (ERAD) or by increasing chaperone activity, the UPR also suppresses global protein synthesis by activating the PERK kinase and by placing the cell in the G2 phase of the cell cycle. The translation of some mRNAs that express proteins required for the ER repair are instead activated by PERK and we have previously demonstrated that PERK-dependent expression of p53/47 induces 14-3-3σ mRNA transcription and is required for G2 arrest. We now show that the increase in 14-3-3σ mRNA levels does not convert into protein expression unless p21 is also downregulated ( Fig. 10 ). Even though phosphorylation of p21 at threonine 57 has been reported to promote G2/M progression by enhancing cyclin B1/CDC2 activity [52] , the T57A and T57D phospho-mutants were equally efficient in suppressing 14-3-3σ expression (data not shown). Thus, inhibition of 14-3-3σ describes a novel p21 function in controlling the cell cycle. In line with this notion, we observed an increase in the amount of phosphorylated CDC2 in the nuclear compartment in the presence of ectopic p21 during ER stress ( Supplementary Fig. 9a ). The best known role of p21 relates to p53 tumour-suppressor activity and G1/S arrest following DNA damage but p21 presents a broad panel of functions, some of which can instead benefit tumour progression [50] , [63] , [64] . The inverse link between p21 and the 14-3-3σ tumour suppressor under certain conditions might help to explain some of these different observations. 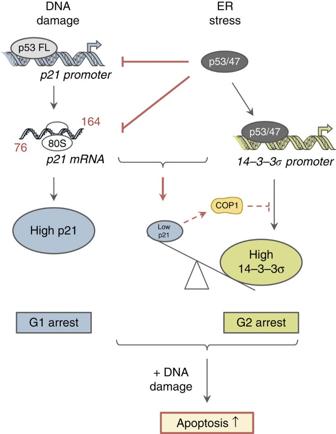Figure 10: Model depicting how p53/47 controls p21 and 14-3-3σ expression to promote G2 arrest during ER stress. Full-length p53 (p53 FL)-dependent transactivation ofp21at the promoter level leads to G1 arrest following DNA damage. ER stress-induced p53/47 triggers14-3-3σmRNA transcription and inhibits p53 FL activity towards thep21promoter. In addition, p53/47 and p53 FL inhibitp21mRNA translation via codons 76–164 of thep21mRNA. This ensures a sufficient suppression of p21 levels to prevent COP1-dependent degradation of 14-3-3σ and thereby allows G2 arrest to facilitate ER stress repair. During ER stress, lowered p21 levels sensitize cells to p53-dependent apoptosis following genotoxic stress. This illustrates a p53-dependent pathway based on the suppression of p21 that dominates during ER stress. Figure 10: Model depicting how p53/47 controls p21 and 14-3-3σ expression to promote G2 arrest during ER stress. Full-length p53 (p53 FL)-dependent transactivation of p21 at the promoter level leads to G1 arrest following DNA damage. ER stress-induced p53/47 triggers 14-3-3σ mRNA transcription and inhibits p53 FL activity towards the p21 promoter. In addition, p53/47 and p53 FL inhibit p21 mRNA translation via codons 76–164 of the p21 mRNA. This ensures a sufficient suppression of p21 levels to prevent COP1-dependent degradation of 14-3-3σ and thereby allows G2 arrest to facilitate ER stress repair. During ER stress, lowered p21 levels sensitize cells to p53-dependent apoptosis following genotoxic stress. This illustrates a p53-dependent pathway based on the suppression of p21 that dominates during ER stress. Full size image Our results show that COP1 is required for p21-dependent regulation of 14-3-3σ but the underlying molecular mechanism for how p21 regulates COP1 activity is unclear. Stabilization of COP1 by the CSN (COP9 signalosome) has been proposed to cause COP1-dependent degradation of 14-3-3σ [35] . However, as p21 does not affect COP1 expression, it is possible that p21 instead regulates the substrate specificity of its E3 ligase activity [42] . This idea is supported by observations that the COP1 substrate JUN, which protects against thapsigargin-induced cell death [65] , is not affected in a p21-dependent manner, whereas the COP1 substrate p53 is ( Fig. 9e and Supplementary Fig. 9b,c ) [41] , [66] . This is also indicative of a feedback loop between p21 and p53 during the UPR via COP1 that needs to be investigated in more details but the observed high p53 levels in p21-null cells, and their repression following p21 re-introduction, are supportive of this notion. Thus, the p21-mediated activation of COP1 that is governed by p53/47 could negatively feedback on p53, similar to the MDM2-p53 feedback loop regulated by full-length p53. ER stress results in a lower amount of phosphorylated ATM following DNA damage, but the activation of ATM downstream targets such as the phosphorylation of p53 is not affected. Hence, the absence of p21 induction during genotoxic and ER stresses is not due to an inhibition of the ATM pathway. The increase in p53-dependent apoptosis following DNA damage in cells undergoing the UPR, further indicates that the ATM pathway remains active during double stress conditions. ATM has been implicated in controlling COP1 activity [67] , but we did not find any support for ATM having a role in p21-dependent control of 14-3-3σ. The role of COP1 in tumorigenesis remains unclear as in vivo studies have identified COP1 as a tumour suppressor, whereas COP1 can also harbour tumour-prone functions in different backgrounds [36] , [37] , [38] , [39] . Our results place COP1 within the ER stress response pathway and should help to better understand the physiological context of COP1 activity, as well as to explain the observation that hypoxia-induced genes are most significantly upregulated in Cop1 -null embryos [36] . This study exemplifies how p53/47 targets an intrinsic G1-G2 regulatory pathway to best serve ER repair and how this impedes on the DNA damage response. p53/47 forms active tetramers more easily [23] and binds to the p21 promoter with higher affinity during the UPR, as compared with its full-length counterpart (see Supplementary Fig. 3b ). As p53/47 lacks the most N-terminal transactivation domain (p53 TA1) it prevents p53 FL-dependent induction of p21 mRNA levels. The neutralization of p53 FL towards the p21 promoter is, nevertheless, not sufficient to reduce p21 protein levels and, most surprisingly, we found that both p53 FL and p53/47 have the capacity to prevent p21 mRNA translation. Our data indicate that this requires transcriptionally active p53 as different mutants with impaired DNA binding activity fail to repress p21. Based on the relative higher levels of p53/47 and its selective activation following ER stress, the suppression of p21 expression appears to be mainly carried out by p53/47 in cells expressing endogenous p53. The inhibition of p21 protein synthesis is mediated by a region of the p21 -CDS that excludes more common mechanisms of translation control that act through the mRNA untranslated regions or p53-regulated miRNAs, and instead favours an RNA structure–protein interaction. The suppression of p21 mRNA translation occurs under all conditions tested, including genotoxic stress. However, the strong induction of p21 gene expression by p53 FL after DNA damage is sufficient to raise p21 protein levels and, thus, the inhibition of p21 synthesis becomes obvious when p21 transcription is suppressed by p53/47 during ER stress. It is interesting that some, but not all, of the steps that lead to activation of 14-3-3σ are ER stress-dependent. For example, the induction of p53/47 and the effect of p21 on 14-3-3σ stability require the ER stress pathway but the effect of p53 on p21 mRNA translation can also take place under normal conditions or during the DNA damage response. An alternative p53 pathway based on the suppression of p21 has broader implications. Arresting cells in G1 plays an important role in allowing cells to repair DNA damage before entering S phase and as ER stress is governed by the tissue microenvironment, the dominant suppression of p21 during the UPR can have adverse effects on how cells protect their genomic integrity and respond to DNA-damaging agents. These results could also offer a molecular explanation for the reported differences in how solid tumours respond to cancer treatments and, thus, help to better predict the efficacy of p53-dependent genotoxic therapies. This notion is supported by observations showing that variations in the p21 levels upon different types of irradiation correlate with the levels of apoptosis and by the link between metabolism, reduced p21 levels and increased DNA damage-induced apoptosis [68] , [69] . The UPR is not restricted to tumours only, as conditions of insufficient perfusion take place in non-cancerous ischemic tissues and the UPR is also associated with neurological disorders, diabetes and inflammation. The expression of p53/47 in normal and tumour tissues has been difficult to estimate as there is no antibody sufficiently specific for this isoform to carry out immunohistochemistry but more recent studies have shown that some tumour types overexpress p53/47 and it will be interesting to determine how this correlates with levels of ER stress and the response to genotoxic treatments [27] . Cell culture p53 wild-type-expressing MLS-1765 (ovarian carcinoma), U2OS (osteosarcoma), MCF-7 (breast adenocarcinoma), A549 (lung carcinoma) and HCT116 (colon carcinoma) or p53-null H1299 (non-small-cell lung carcinoma) and Saos-2 (osteosarcoma) human cell lines were used. MLS-1765 cells were given by Professor P. Åman (University of Gothenburg, Gothenburg, Sweden) and HCT116 cells were kindly provided by Professor B. Vogelstein (Johns Hopkins University, Baltimore, MD, USA). Other cell lines were purchased from American Type Culture Collection. MLS-1765, H1299 and Saos-2 cells were cultured in RPMI 1640 medium (no glutamine); U2OS and HCT116 cells in McCoy’s 5A medium (modified, GlutaMAX) and MCF-7 and A549 cells in Dulbecco’s modified Eagle’s medium medium (high glucose, no glutamine). All media (Invitrogen) were supplemented with 10% fetal bovine serum, 2 mM L -glutamine, 100 U ml −1 penicillin and 100 μg ml −1 streptomycin (Invitrogen) except McCoy’s 5A where no L -glutamine was added. Cell lines were maintained at 37 °C in a humidified 5% CO 2 incubator. All experiments were performed using exponentially growing cells and cell counts were carried out using a Malassez hemocytometer. Cell transfection and treatment Twenty-four hours before transfection, 2 × 10 5 cells were seeded in six-well plates (or 4 × 10 5 cells in 6 cm diameter plates for inhibition of protein synthesis, inhibition of proteasomal degradation or metabolic pulse labelling). cDNA transfections were made using GeneJuice reagent (EMD Chemicals) as per manufacturer’s protocol. Total amount of DNA was kept constant by addition of empty vector. After 8 h, medium was replaced for siRNA transfection. siRNAs targeting p21 , COP1 or p53 and AllStars negative control siRNA were from Qiagen and transfected using HiPerFect reagent (Qiagen) following manufacturer’s instructions. Efficiency of siRNAs was assessed by RT–qPCR and western blot analysis (see Supplementary Fig. 10 and figures where siRNA was used). Cells were further incubated for 24 h before treatment. Drugs’ stock solutions were prepared in DMSO (Euromedex) unless specified otherwise and cells were treated with 100 nM thapsigargin, 7.5 μg ml −1 tunicamycin, 100 nM Dox (Sigma-Aldrich) or 0.1% DMSO for 16 h. For investigating the DNA damage response during UPR activation, cells were subjected to 1 μM Dox during the last hours of thapsigargin or DMSO treatment as follows: HCT116, 1 h Dox pulse followed by 2 h incubation in drug-free medium; A549, 1 h Dox pulse followed by 4 h in drug-free medium; H1299, 2 h Dox pulse and Saos-2, 2 h Dox pulse followed by 2 h in drug-free medium. These time points were determined as optimal for S1981-pATM, p53 and p21 levels induction by Dox alone in each cell line and were kept for all experimental points in corresponding western blots and apoptosis assays (in Fig. 1 and Supplementary Fig. 1 ). Inhibition of protein synthesis was performed by treating cells with 5 μg ml −1 cycloheximide (EMD Chemicals, stock solution prepared in 30% ethanol) for 0 to 6 h during the last hours of thapsigargin treatment. Inhibition of proteasomal degradation was achieved by treating cells with 5 μM epoxomicin (Peptide Institute) during the last 2 h of thapsigargin treatment. The MLN4924 small-molecule inhibitor of Nedd8-activating enzyme was a kind gift from Dr C.J. Hastie (Medical Sciences Institute, Dundee, Scotland, UK) and was used at 3 μM for 4 h in the culture medium. ATM inhibitor (EMD Biosciences) was used at 10 μM for 20 h. Expression vectors All constructs were in pcDNA3 unless otherwise indicated. p53 wt, p53 FL and p53/47 constructs have been described previously [23] and are schematically represented (see Fig. 2a ). p21, 3X FLAG-p21 and COP1 were kind gifts from Dr E. Worrall (University of Edinburgh, Scotland, UK). 3X FLAG-p21 was modified as follows: initiation codon for p21 was deleted and STOP codon was added at the end of the p21-CDS. Resulting 3X FLAG-p21 was subcloned into pcDNA3. COP1 wild-type sequence (not pcDNA3) was restored by site-directed mutagenesis (H626N). 14-3-3σ was generated from pcDNA3-HA 14-3-3 sigma, from Pr. M. Yaffe (Massachusetts Institute of Technology, Cambridge, MA, USA) by removal of HA tag sequence and addition of initiation and STOP codons. Site-directed mutagenesis was performed to create p21 S130A mutant and DNA-binding mutations R175H, R248W and R273H in each of the p53 constructs. p16 CDS was amplified and subcloned into pcDNA3. p21 -Luc in pGL3-Basic vector encodes the firefly luciferase under the control of p21 promoter and was a kind gift from Dr M. Sabbah (Saint Antoine Hospital, Paris, France). pRL-TK encoding the Renilla reniformis luciferase under HSV-thymidine kinase weak promoter was purchased from Promega. The p21 mRNA CDS-EGFP reporter constructs were made as follows: p21 CDS was amplified from the above-mentioned p21-encoding construct without initiation and STOP codons and inserted in front of the EGFP open reading frame in the pEGFP-N1 vector. The two in-frame p21 AUGs were sequentially substituted with alanine by site-directed mutagenesis to suppress expression of fusion products and all three reporter constructs are schematically represented (see Fig. 5b ). Deletion mutants of the p21 CDS were created from the reporter construct that carry alanine substitutions for both in-frame p21 AUGs (C). For deletion mutants containing codons 28-164, 76-164, 2-90, 91-164 and 2-75, the sequence of interest was PCR-amplified and subcloned into pEGFP-N1. To delete codons 76-90 (deletion mutant 2-75; 91-164), overlap extension method was used and the final amplicon was subcloned into pEGFP-N1. All deletion mutants are schematically represented (see Fig. 5d ). Western blotting Cells were lysed in buffer (20 mM HEPES KOH pH 7.5, 50 mM β-glycerophosphate, 1 mM EDTA pH 8.0, 1 mM EGTA pH 8.0, 0.5 mM Na 3 VO 4 , 100 mM KCl, 10% glycerol and 1% Triton X-100) supplemented with complete protease inhibitor cocktail (Roche Diagnostics). Protein concentration was determined using Bradford (Bio-Rad) and equal protein amounts were separated by 15% SDS–polyacrylamide gel electrophoresis. After electrophoretic transfer to BioTrace NT pure nitrocellulose blotting membrane (PALL), membranes were blocked with 5% non-fat dry milk in Tris-buffered saline pH 7.6 containing 0.1% Tween-20. Proteins were probed by overnight incubation at 4 °C with the following antibodies. Anti-p53 Bp53-10.1 and anti-Hsp90α+β mouse monoclonal antibodies (mAbs), as well as anti-p53 CM-1 and ACMDD rabbit polyclonal antibodies (pAbs) were kindly provided by Dr B. Vojtesek, (Masaryk Memorial Cancer Institute, Brno, Czech Republic). For the ACMDD sera raised against the N-terminus of p53/47 and used where indicated, the membranes were pre-incubated with 0.4% paraformaldehyde at room temperature for 1 h and washed before blocking. Anti-p21 (12D1) and anti-phospho-CDC2 (Tyr15) rabbit mAbs, anti-phospho-p53 (Ser15), anti-cleaved PARP and anti-PARP rabbit pAbs as well as anti-CDC2 mouse mAb were from Cell Signaling Technology; anti-14-3-3σ (CS112-2A8) and anti-phospho-ATM (Ser1981) mouse mAbs from Millipore; anti-ATM mouse mAb from Genetex; anti-caspase 7 mouse mAb from BD Pharmingen; anti-BiP rabbit pAb, anti-p16 (DCS50.1) and anti-CHOP mouse mAbs from Abcam; anti-COP1 rabbit Ab from Bethyl Laboratories; anti-JUN mouse Ab from BD Biosciences; anti-calreticulin from Stressgen; anti-calnexin mouse mAb from Calbiochem; and anti-tubulin, anti-β-actin and anti-FLAG M2 mouse mAbs from Sigma-Aldrich. Membranes were then incubated with appropriate HRP-conjugated secondary antibodies (Dako) and detection was performed using ECL and Hyperfilm (Amersham). For quantification of protein bands, chemiluminescence images were acquired using CHEMI-SMART 5000 documentation system and Chemi-Capt software (Vilbert Lourmat), and densitometry analysis was performed with Bio-PROFIL Bio 1-D software (Vilbert Lourmat). Uncropped images of the more important western blots are provided in the Supplementary Information ( Supplementary Figs 11–13 ). Cell cycle analysis and apoptosis assay For cell cycle distribution, cells were fixed by overnight incubation in ice-cold 70% ethanol. After 30 min incubation with 100 U ml −1 RNase A (Sigma-Aldrich) at 37 °C, cells were stained with 10 μg ml −1 propidium iodide (PI, Sigma-Aldrich). For apoptosis assay, both floating and attached cells were collected 18 h following DMSO or thapsigargin treatment for HCT116, 24 h for H1299 and Saos-2. Cells were then simultaneously stained with Annexin V-FITC and PI using the Annexin V-FITC Apoptosis Detection Kit from Sigma-Aldrich, as per manufacturer’s instructions. Annexin V binds to exposed phosphatidylserines on early apoptotic cells, whereas the non-vital dye PI stains late apoptotic and necrotic cells. FACS was performed for 50,000 events using BD FACSCanto II flow cytometer and analysis was carried out with BD FACSDiva software. RNA extraction, reverse transcription and RT–qPCR Total RNA was extracted with RNeasy Mini Kit (Qiagen) following manufacturer’s instructions. cDNA synthesis was carried out using the Moloney murine leukaemia virus reverse transcriptase and Oligo(dT) 12-18 Primer (Invitrogen). RT–qPCR was performed on StepOne real-time PCR system (Applied Biosystems) using TaqMan Gene Expression Master Mix and Assays for p21 , 14-3-3σ and actin (Applied Biosystems). Assays for p21 and 14-3-3σ are localized within the mRNA-CDS and thus allow detection of both endogenous and exogenous mRNA levels. The relative abundances of p21 and 14-3-3σ mRNAs were calculated after normalization to the corresponding actin levels. RT–qPCR for p53 , BiP and GAPDH was performed using Perfecta SYBR Green FastMix, ROX (Quanta Biosciences) and the following primers: p53 forward 5′-TGGGCTTCTTGCATTCTG-3′; p53 reverse 5′-GCTGTGACTGCTTGTAGATGGC-3′; BiP forward 5′-GCAACCAAAGACGCTGGAACT-3′; BiP reverse 5′-CCTCCCTCTTATCCAGGCCATA-3′; GAPDH forward 5′-GAGTCAACGGATTTGGTCGT-3′ and GAPDH reverse 5′-GACAAGCTTCCCGTTCTCAG-3′. For ChIP assays, Perfecta SYBR Green FastMix, ROX (Quanta Biosciences) was used and region of the p21 promoter was amplified using the following primers: forward 5′-GTGGCTCTGATTGGCTTTCTG-3′ and reverse 5′-CTGAAAACAGGCAGCCCAAG-3′. Its relative abundance was calculated after normalization to the input GAPDH levels, detected with primers forward 5′-TACTAGCGGTTTTACGGGCG-3′ and reverse 5′- TCGAACAGGAGCAGAGAGCGA-3′. Dual luciferase assay 8 × 10 4 cells were seeded in 12-well plates. p21 -Luc vector and pRL-TK (internal control reporter vector) were co-transfected with indicated p53 constructs. Cells were lysed in passive lysis buffer (Promega) and lysates were distributed to a white 96-well plate OptiPlate-96 (Perkin-Elmer). Promoter activity was simultaneously measured on FLUOstar Optima luminometer (BMG Labtech) using the Dual-Luciferase Reporter Assay System (Promega) as per manufacturer’s protocol. The relative change in the activity of the p21 promoter was calculated after normalization to the corresponding pRL-TK activity. Metabolic radiolabelling and immunoprecipitation Cells were kept at 37 °C, 5% CO 2 in Dulbecco’s modified Eagle’s starvation medium (without methionine, cystine and L -glutamine, Sigma-Aldrich) supplemented with 2% dialysed fetal bovine serum, 2 mM L -glutamine, 100 U ml −1 penicillin and 100 μg ml −1 streptomycin, together with 5 μM of the proteasome inhibitor epoxomicin during the last 2 h of DMSO or thapsigargin treatment. Cells were metabolically radiolabelled with 45 μCi ml −1 of EasyTag Express 35S-methionine Protein Labeling Mix (Perkin-Elmer) for the last 30 min. Cells were lysed in buffer (20 mM Tris-HCl, pH 7.5, 150 mM NaCl and 1% NP-40) supplemented with complete protease inhibitor cocktail. Equal protein amounts, as determined by Bradford, were pre-cleared with mouse serum (Dako) and protein G sepharose bead slurry (Sigma-Aldrich). Samples were immunoprecipitated by overnight incubation with anti-p21 mouse DCS60 mAb (Cell Signaling Technology) or non-specific mouse IgG antibody (Jackson ImmunoResearch Laboratories) at 4 °C. Bead slurry was added and samples incubated for 4 h at 4 °C. Beads were washed and boiled in 2 × Laemmli buffer. Proteins were resolved in 15% SDS–polyacrylamide gel electrophoresis, followed by fixation in 7% methanol and 21% acetic acid, amplification in Amplify (Amersham) and drying of the gels. Detection was achieved by exposure to X-ray film. Autoradiography of input samples confirmed equal incorporation of overall 35 S-methionine into cellular proteins. For quantification of immunoprecipitated radiolabelled proteins, gels were exposed to phosphor imager screen, scanned using a Storm 840 phosphorimager (Molecular Dynamics) and analysed with ImageQuant software (Molecular Dynamics). ChIP Cells were cross-linked with 1% formaldehyde for 10 min at 37 °C and reaction was quenched using 1 M glycine (5 min, 37 °C). Cells were lysed in RIPA lysis buffer supplemented with complete protease inhibitor cocktail and sonicated. Lysates were pre-cleared with rabbit serum (Dako) and protein G sepharose bead slurry. Samples were immunoprecipitated by overnight incubation with anti-p53 rabbit CM-1 pAb at 4 °C. Bead slurry was added and samples incubated for 4 h at 4 °C. Beads were washed and cross-link was reversed by overnight incubation at 65 °C. Proteinase K (Sigma) was added for 1 h at 45 °C and DNA was purified using QIAquick (Qiagen) for RT–qPCR analysis. Statistical analysis Data shown are mean±s.d. of minimum three independent experiments. Two-tailed unpaired Student’s t -test was performed by comparing data to the corresponding reference point or as indicated and P values are shown. * P <0.05; ** P <0.01; *** P <0.001, NS, not significant. How to cite this article: Mlynarczyk, C. and Fåhraeus, R. Endoplasmic reticulum stress sensitizes cells to DNA damage-induced apoptosis through p53-dependent suppression of p21 CDKN1A . Nat. Commun. 5:5067 doi: 10.1038/ncomms6067 (2014).